α-SNAP inhibits AMPK signaling to reduce mitochondrial biogenesis and dephosphorylates Thr172 in AMPKαin vitro The AMP-activated protein kinase (AMPK) regulates metabolism in normal and pathological conditions and responds to nutrients, hormones, anti-diabetic drugs and physical exercise. AMPK is activated by the kinase LKB1 and inactivated by phosphatases whose identities remain uncertain. Here we show that AMPK associates with α-SNAP, an adapter that enables disassembly of cis-SNARE complexes formed during membrane fusion. Knockdown of α-SNAP activates AMPK to phosphorylate its endogenous substrates acetyl CoA carboxylase and Raptor, and provokes mitochondrial biogenesis. AMPK phosphorylation is rescued from α-SNAP RNA interference by LKB1 knockdown or expression of wild-type but not mutated α-SNAP. Recombinant wild-type but not mutated α-SNAP dephosphorylates pThr172 in AMPKα in vitro . Overexpression of wild-type but not mutated α-SNAP prevents AMPK activation in cells treated with agents to elevate AMP concentration. The mouse α-SNAP mutant hyh (hydrocephalus with hop gait) shows enhanced binding and inhibition of AMPK. By negatively controlling AMPK, α-SNAP therefore potentially coordinates membrane trafficking and metabolism. Cellular energy in the form of ATP drives biosynthetic pathways and supports essential processes such as ion transport, cytoskeletal integrity and membrane trafficking [1] , [2] . Homeostasis requires throttling these demands for energy while regenerating ATP, predominantly by mitochondrial respiration. Central to this balancing act is the 5′-adenosine monophosphate (AMP)-activated protein kinase (AMPK), an enzyme comprised of catalytic α subunit plus regulatory β and γ subunits, the latter of which alternatively binds ATP, ADP or AMP to gauge metabolic status [1] , [2] . In terms of animal physiology, AMPK is a critical node of regulation, for it controls fat and carbohydrate metabolism, and responds to nutrients, hormones, drugs and physical exercise in both normal and pathological conditions [3] . The rise in ratio of [AMP+ADP] versus [ATP] because of energy expenditure or inhibition of respiration activates AMPK predominantly by phosphorylation of T172 in the kinase activation loop in the α subunit [4] . The pT172 levels depend on a balance between the primary AMPK activating kinase LKB1 [5] , [6] and dephosphorylation by protein phosphatases [7] . Dephosphorylation of pT172 is affected by AMP and ADP [8] , [9] , however, the identity of the physiologically relevant AMPK phosphatase(s) remains unclear. Here, we discovered that inactive AMPK bound to ATP stably associates with the protein alpha-soluble N- ethylmalemide sensitive factor attachment protein (α-SNAP) that acts as a negative regulator of the kinase. Knockdown of α-SNAP resulted in enhanced phosphorylation of T172 in AMPK, phosphorylation of AMPK substrates and increased mitochondrial biogenesis and respiration. Effects of α-SNAP knockdown were rescued by overexpression of α-SNAP and complemented by knockdown of LKB1, showing the effects were due to T172 phosphorylation. Furthermore, recombinant α-SNAP dephosphorylated AMPK in vitro , even though the sequence and structure of α-SNAP does not resemble any known protein phosphatase. Mutations in α-SNAP are shown to provide either loss-of-function or gain-of-function phenotypes relative to AMPK inactivation. Multiple actions of α-SNAP provide a connection between membrane fusion events and metabolism required to fuel these processes. Binding of AMPK to α-SNAP is responsive to ATP To explore regulation of AMPK we immunoprecipitated FLAG-tagged AMPK-γ1 from stably transfected HEK293 cells. Silver staining after SDS–PAGE revealed the AMPKγ subunit co-precipitated endogenous α and β subunits, with or without oligomycin addition to the cells to activate AMPK ( Fig. 1a ). In addition, a 35 kDa protein associated with inactive (lane 2), but not active AMPK (lane 3). This band was excised and liquid chromatography-coupled tandem mass spectrometry/mass spectrometry identified it as α-SNAP ( a.k.a. NAPA; NSF attachment protein, alpha). For many years α-SNAP has been studied as factor required for activation of the NSF ATPase for resolution of cis-SNARE (SNAP receptor) complexes formed during membrane fusion [10] . The activity of NSF allows repeated rounds of membrane fusion, therefore α-SNAP regulates a critical limiting step in intracellular membrane trafficking and exocytosis [11] . We confirmed the association of α-SNAP with AMPK by immunoprecipitation of endogenous α-SNAP with endogenous AMPK that was recovered from unstressed cells ( Fig. 1b ). Addition of 2-deoxyglucose or phenformin metabolically stressed cells and elevated [AMP]-activated AMPK, evident from the increase in phosphorylation of T172 in AMPKα and robust phosphorylation of S79 in the endogenous AMPK substrate, acetyl CoA carboxylase (ACC). Activation of AMPK substantially decreased its co-immunoprecipitation with endogenous α-SNAP ( Fig. 1b ). This reduced binding to AMPK in cells with elevated [AMP] indicated that association with α-SNAP did not depend on the phosphorylation of T172 in AMPK, but was sensitive to the conformation of the kinase. Co-expression of HA-α-SNAP with FLAG-AMPKαβγ allowed reciprocal anti-HA or anti-FLAG co-precipitation of the proteins ( Fig. 1c . ), even though artificial binding can occur because of overexpression of proteins. We think that α-SNAP contacts AMPK at multiple sites, in different subunits of the heterotrimer, just as α-SNAP simultaneously binds both NSF and SNARE proteins [11] . 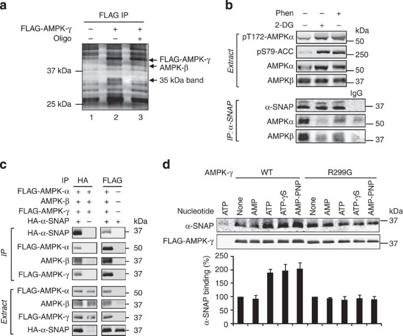Figure 1: α-SNAP associates with AMPK bound to ATP. (a) HEK293 cells as control (lane 1) and cells stably expressing FLAG-AMPKγ1 were treated for 20 min with vehicle (lane 2) or 2 μM oligomycin (oligo) (lane 3). AMPK was isolated by FLAG immunoprecipitation (IP) and proteins resolved by SDS–PAGE, followed by silver staining. The AMPK β and γ subunits (lane 2 and 3) are marked with arrows, and the prominent 35 kDa band (lane 2) was excised and analysed by LC/MS/MS mass spectrometry. (b) Immunoblots of cell extracts (upper panels) and immunoprecipitates (IP, lower panels) of endogenous α-SNAP, compared with non-specific IgG as a control. HEK293T cells were untreated as control or treated with 25 mM 2-deoxyglucose (2-DG), or 3 mM phenformin (phen). (c) FLAG-AMPKα2, β1, γ1 were co-expressed with HA-α-SNAP in HEK293T cells. Cell extracts and HA and FLAG immunoprecipitates were immunoblotted. (d) FLAG-AMPKγ1 wild-type (WT) and R299G were expressed in HEK293T cells and recovered on beads as FLAG immunoprecipitates. Beads were incubated with purified recombinant α-SNAP protein without or with addition of the indicated nucleotides. Samples were immunoblotted and staining intensity normalized relative to samples with no nucleotide added. Data represent means±s.e.m. forn=3 and statistical analysis of ANOVA followed by multiple Fisher’s test was performed (WT NONE versus ATP, ATP-γS and AMP-PNP:P<0.02; WT NONE versus AMP:P=0.997; R299G variant,P=0.927). Figure 1: α-SNAP associates with AMPK bound to ATP. ( a ) HEK293 cells as control (lane 1) and cells stably expressing FLAG-AMPKγ1 were treated for 20 min with vehicle (lane 2) or 2 μM oligomycin (oligo) (lane 3). AMPK was isolated by FLAG immunoprecipitation (IP) and proteins resolved by SDS–PAGE, followed by silver staining. The AMPK β and γ subunits (lane 2 and 3) are marked with arrows, and the prominent 35 kDa band (lane 2) was excised and analysed by LC/MS/MS mass spectrometry. ( b ) Immunoblots of cell extracts (upper panels) and immunoprecipitates (IP, lower panels) of endogenous α-SNAP, compared with non-specific IgG as a control. HEK293T cells were untreated as control or treated with 25 mM 2-deoxyglucose (2-DG), or 3 mM phenformin (phen). ( c ) FLAG-AMPKα2, β1, γ1 were co-expressed with HA-α-SNAP in HEK293T cells. Cell extracts and HA and FLAG immunoprecipitates were immunoblotted. ( d ) FLAG-AMPKγ1 wild-type (WT) and R299G were expressed in HEK293T cells and recovered on beads as FLAG immunoprecipitates. Beads were incubated with purified recombinant α-SNAP protein without or with addition of the indicated nucleotides. Samples were immunoblotted and staining intensity normalized relative to samples with no nucleotide added. Data represent means±s.e.m. for n =3 and statistical analysis of ANOVA followed by multiple Fisher’s test was performed (WT NONE versus ATP, ATP-γS and AMP-PNP: P <0.02; WT NONE versus AMP: P =0.997; R299G variant, P =0.927). Full size image Purified, recombinant α-SNAP bound directly to FLAG-AMPKγ in an in vitro assay and binding was enhanced by addition of ATP ( Fig. 1d ). AMPK is allosterically regulated by binding of either ATP or AMP/ADP to the γ subunit, at sites formed by four cystathionine beta synthase domains [3] . The assay revealed a two-fold increase in binding to AMPKγ in the presence of ATP or non-hydrolyzable derivatives of ATP. In contrast, there was no ATP-dependent increase in α-SNAP binding with FLAG-AMPKγ R299G (equivalent to R531G in γ2), a single residue substitution in the cystathionine beta synthase4 domain that is linked to human Wolf–Parkinson–White cardiomyopathy and known to affect nucleotide binding [12] . We concluded that α-SNAP preferentially interacts with the ATP-bound conformation of the γ subunit, which would account for the differential co-immunoprecipitation from cells, depending on metabolic stress-induced increases in [AMP]. AMPK phosphorylation at T172 is negatively regulated by α-SNAP We knocked down α-SNAP in cells by RNA interference (RNAi) using two different sequences of short hairpin RNAs (shRNA) and examined effects on AMPK phosphorylation and signalling ( Fig. 2 ). Both of these shRNA effectively reduced α-SNAP to low levels and resulted in a significant 4 to 5-fold increase in phosphorylation of T172 in AMPK, relative to controls expressing shRNA for a sequence in GFP ( Fig. 2a ). Knockdown of α-SNAP significantly increased phosphorylation of S79 in ACC and S792 in Raptor, an essential subunit of the mTORC1 complex, showing activation of AMPK led to phosphorylation of its endogenous substrates to suppress anabolic metabolism. Phosphorylation of Raptor S792 negatively regulates mTORC1 activity [13] , and indeed phosphorylation of T389 in the mTORC1 substrate p70S6K was reduced by knockdown of α-SNAP ( Fig. 2a ). As an additional control we used RNAi to knockdown NSF, the known partner of α-SNAP. Knockdown of NSF did not affect the basal phosphorylation of AMPKα, activation of AMPK by 2-deoxyglucose or AMPK signalling to endogenous ACC, Raptor and p70S6K ( Fig. 2a ). Therefore, activation of AMPK signalling in response to knockdown of α-SNAP was not secondary to NSF-dependent actions in cells. Activation of AMPK due to knockdown of α-SNAP was not secondary to elevation of the [AMP+ADP]/[ATP] nucleotide ratio. Knockdown of α-SNAP actually reduced the cellular ratio of [AMP+ADP]/[ATP] ( Supplementary Table S1 ). On the other hand, overexpression of α-SNAP significantly blunted the activation of AMPK by metabolic stress induced by oligomycin, phenformin or 2-deoxyglucose relative to controls, and reduced AMPK-dependent signalling to ACC and Raptor ( Fig. 2b ). These results showed α-SNAP imposes a major inhibitory restraint on AMPK activation and anabolic signalling in living cells. 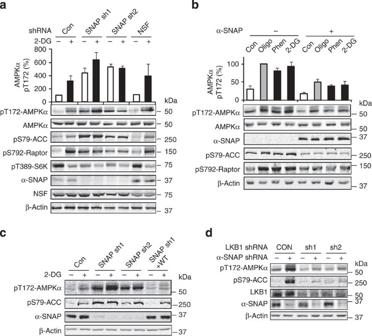Figure 2: α-SNAP negatively regulates AMPK signalling in living cells. (a) HEK293T cells expressing lentiviral shRNA targeting GFP (control, CON), α-SNAP (SNAP sh1 and sh2), or NSF were treated +/− 25 mM 2-deoxyglucose (2-DG) for 20 min and cell extracts analysed by immunoblotting, with AMPKα and β-actin as loading controls. Data represent means±s.e.m. forn=3 and statistical analysis of ANOVA followed by multiple Fisher’s test was performed (basal CON versus basal α-SNAP sh1, sh2:P<0.001; basal CON versus basal NSF sh:P=0.903). (b) HEK293T cells were transfected in 6-well plates for 36 h with empty vector or vector expressing α-SNAP. Cells were treated with 2 μM oligomycin (oligo), 3 mM phenformin (phen) or 25 mM 2-DG for 20 min and cell extracts analysed by immunoblotting, with AMPKα and β-actin as loading controls. Data represent means±s.e.m. forn=3 and statistical analysis of two-way ANOVA test was performed (without versus with α-SNAP expression:P<0.001). (c) Madin–Darby canine kidney (MDCK) cells were infected with lentivirus encoding shRNA targeting GFP (CON), dog α-SNAP (SNAP sh1 and sh2) or SNAP sh1 together with expression vector for human α-SNAP. Cells were treated (−/+) with 25 mM 2-DG for 20 min and cell extracts analysed by immunoblotting. (d) HEK293T cells were knocked down by infection with lentiviral shRNA targeting GFP (CON) or LKB1 (sh1 and sh2). Cells were subsequently infected with lentiviral shRNA targeting GFP (−) or α-SNAP sh1 (+) and extracts analyzed by immunoblotting. Figure 2: α-SNAP negatively regulates AMPK signalling in living cells. ( a ) HEK293T cells expressing lentiviral shRNA targeting GFP (control, CON), α-SNAP (SNAP sh1 and sh2), or NSF were treated +/− 25 mM 2-deoxyglucose (2-DG) for 20 min and cell extracts analysed by immunoblotting, with AMPKα and β-actin as loading controls. Data represent means±s.e.m. for n =3 and statistical analysis of ANOVA followed by multiple Fisher’s test was performed (basal CON versus basal α-SNAP sh1, sh2: P <0.001; basal CON versus basal NSF sh: P =0.903). ( b ) HEK293T cells were transfected in 6-well plates for 36 h with empty vector or vector expressing α-SNAP. Cells were treated with 2 μM oligomycin (oligo), 3 mM phenformin (phen) or 25 mM 2-DG for 20 min and cell extracts analysed by immunoblotting, with AMPKα and β-actin as loading controls. Data represent means±s.e.m. for n =3 and statistical analysis of two-way ANOVA test was performed (without versus with α-SNAP expression: P <0.001). ( c ) Madin–Darby canine kidney (MDCK) cells were infected with lentivirus encoding shRNA targeting GFP (CON), dog α-SNAP (SNAP sh1 and sh2) or SNAP sh1 together with expression vector for human α-SNAP. Cells were treated (−/+) with 25 mM 2-DG for 20 min and cell extracts analysed by immunoblotting. ( d ) HEK293T cells were knocked down by infection with lentiviral shRNA targeting GFP (CON) or LKB1 (sh1 and sh2). Cells were subsequently infected with lentiviral shRNA targeting GFP (−) or α-SNAP sh1 (+) and extracts analyzed by immunoblotting. Full size image We observed similar effects of α-SNAP knockdown on AMPK phosphorylation and signalling in a second cell line, Madin–Darby Canine Kidney epithelial cells. Knockdown of α-SNAP using canine shRNA elevated the level of pT172 in AMPK, and increased phosphorylation of ACC at S79 in both unstimulated cells and cells treated with 2-deoxyglucose ( Fig. 2c ). The increased phosphorylation of AMPK and ACC due to knockdown of α-SNAP was reduced to levels in control cells by stable expression of human α-SNAP that was not targeted by canine shRNA ( Fig. 2c ). Furthermore, increased phosphorylation of AMPK and ACC in response to α-SNAP knockdown was suppressed by the coincident knockdown of LKB1 using either of two independent shRNA sequences ( Fig. 2d ). The requirement for the AMPK activating kinase LKB1 for activation of AMPK showed that α-SNAP was controlling phosphorylation of T172. Knockdown of α-SNAP enhances oxygen consumption and mitochondrial biogenesis To gauge the physiological and metabolic effects of α-SNAP knockdown we used the Seahorse analyser to measure the cellular oxygen consumption rate (OCR). Knockdown of α-SNAP significantly elevated the OCR over the control ( Fig. 3a ), and LKB1 knockdown itself did not alter the OCR but did prevent the increase in OCR due to α-SNAP knockdown, showing the responses involved regulation of AMPK. As controls, in time course experiments, the addition of complex V inhibitor oligomycin reduced and complex I inhibitor rotenone fully extinguished the OCR and conversely, FCCP as an uncoupler of oxidative-phosphorylation increased the OCR ( Fig. 3b ). In contrast, the extracellular acidification rate (ECAR), an indicator of anaerobic glycolytic lactate production, did not change significantly in α-SNAP knockdown cells relative to controls ( Supplementary Fig. S1a ). AMPK is known to induce mitochondrial biogenesis via PGC-1α and SIRT1 [14] . We quantified mitochondrial biogenesis by citrate synthase activity and quantitative immunoblotting for mitochondrial proteins such as ATP synthase, complex III and cytochrome oxidase subunit IV. Knockdown of α-SNAP by either of two shRNA-activated AMPK and significantly increased mitochondrial biogenesis ( Fig. 3c and Supplementary Fig. S1b ). The increase in mitochondrial content was suppressed by knockdown of LKB1, by either of two independent shRNA ( Fig. 3e and Supplementary Fig. S1c ). This showed that the responses to α-SNAP knockdown depended on the phosphorylation of T172 in AMPK. 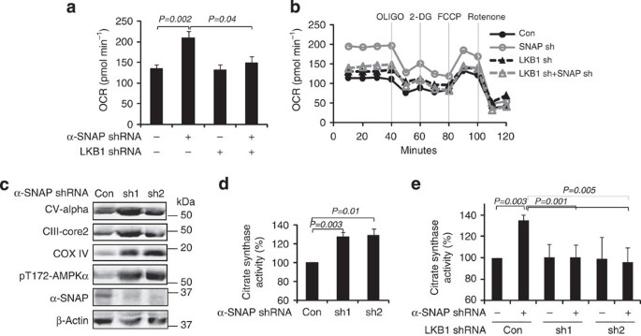Figure 3: Knockdown of α-SNAP elevates mitochondrial respiration and stimulates mitochondrial biogenesis. (a) OCR (pmol/min) in HEK293T cells measured by a Seahorse Analyser. Lentiviral shRNA infected cells are indicated and double knockdown was performed asFig. 2d. Basal measurements were normalized for protein concentrations and the mean±s.e.m. from four independent experiments are plotted. Student’st-test was used to calculate significance. (b) Seahorse continuous measurement of OCR. (c) HEK293T cells were infected with lentiviral shRNA targeting GFP (control, CON) or α-SNAP (SNAP sh1 and sh2). Mitochondrial proteins were detected by immunoblotting: CV-α, ATP synthase subunit alpha; CIII-core2, Complex III subunit Core 2; COXIV, cytochrome c oxidase subunit IV. (d,e) Citrate synthase activity as a measure of mitochondrial content was assayed and normalized relative to controls. Data represent mean±s.e.m. (n=4) andP-values from Student’st-test of significance are indicated. (d) Cells prepared as (c). (e) α-SNAP and LKB1 were knocked down as described inFig. 2d. Figure 3: Knockdown of α-SNAP elevates mitochondrial respiration and stimulates mitochondrial biogenesis. ( a ) OCR (pmol/min) in HEK293T cells measured by a Seahorse Analyser. Lentiviral shRNA infected cells are indicated and double knockdown was performed as Fig. 2d . Basal measurements were normalized for protein concentrations and the mean±s.e.m. from four independent experiments are plotted. Student’s t- test was used to calculate significance. ( b ) Seahorse continuous measurement of OCR. ( c ) HEK293T cells were infected with lentiviral shRNA targeting GFP (control, CON) or α-SNAP (SNAP sh1 and sh2). Mitochondrial proteins were detected by immunoblotting: CV-α, ATP synthase subunit alpha; CIII-core2, Complex III subunit Core 2; COXIV, cytochrome c oxidase subunit IV. ( d , e ) Citrate synthase activity as a measure of mitochondrial content was assayed and normalized relative to controls. Data represent mean±s.e.m. ( n =4) and P- values from Student’s t -test of significance are indicated. ( d ) Cells prepared as ( c ). ( e ) α-SNAP and LKB1 were knocked down as described in Fig. 2d . Full size image α-SNAP dephosphorylates T172 in AMPK in vitro How does α-SNAP reduce AMPK activation? The T172 site in AMPKα is phosphorylated by LKB1, which is thought to be a constitutively active AMPK kinase [15] . Therefore, we reasoned that α-SNAP was promoting dephosphorylation of AMPK, either as an adapter recruiting a protein Ser/Thr phosphatase, or alternatively α-SNAP could have phosphatase activity. To test this latter idea we expressed four versions of recombinant α-SNAP in bacteria and purified the proteins to homogeneity ( Fig. 4a ). These were (1) wild-type (WT), (2) the hyh mutant M105I, (3) L294A, (substitution of the only strictly conserved residue in the C-terminal of SNAPs) and (4) α-SNAP (1–285) deleted of the C-terminal 10 residues. Previous studies showed the L294A and 1–285 mutants of α-SNAP bound to NSF the same as wild-type, but did not activate NSF and therefore acted as dominant-negative proteins in cells, blocking resolution of SNARE complexes and exocytosis [16] . We found that recombinant WT α-SNAP but not L294A or 1–285 exhibited phosphatase activity with the chemical substrate DiFMUP and pSer/pThr peptides (unpublished data). We measured in vitro dephosphorylation of AMPK recombinant protein by purified WT α-SNAP ( Fig. 4b ). GST-AMPKα (1–392) was purified from bacteria and 32 P-labelled at T172 with purified CaMKK II for use as substrate. The phosphatase reaction was visualized by the loss of 32 P from the acid precipitated substrate recovered from the assay ( Fig. 4b ). The release of 32 P from this substrate showed a linear concentration dependence on the amount of α-SNAP added to the assay ( Fig. 4c ). The specific activity was calculated as 24.9 pmol phosphate released per min per μg enzyme, within the range of other known protein phosphatases. In addition, we assayed the four different forms of recombinant α-SNAP for dephosphorylation of pT172 in AMPKα that was immunoprecipitated from extracts of stimulated cells. Both the WT and M105I α-SNAP efficiently and completely dephosphorylated T172 in AMPK, but neither the L294A nor 1–285 mutant of α-SNAP dephosphorylated AMPK under the same conditions ( Fig. 4d ). As a test for substrate specificity, we compared pT308 in Akt and pS792 in Raptor as alternative phosphoprotein substrates in the assay with recombinant WT α-SNAP, but these proteins were not dephosphorylated ( Fig. 4e ). The results showed that α-SNAP could act as a protein phosphatase in biochemical in vitro assays to dephosphorylate T172 in AMPK. 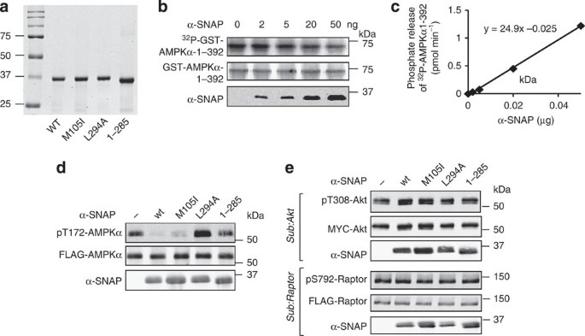Figure 4: α-SNAP dephosphorylates pT172 in AMPKα. (a) Coomassie blue staining of purified wild-type (WT) α-SNAP, mutants M105I, L294A and 1–285 were purified, used in assays for phosphatase activity. (b,c)32P-labeled GST-AMPKα1–392 recombinant protein was used as substrate of α-SNAP phosphatase. α-SNAP (2, 5, 10 and 50 ng) was incubated with32P-GST-AMPKα-1–392. (b)32P-GST-AMPKα-1–392 recovered by trichloroacetic acid precipitation was resolved in SDS–PAGE and detected by phosphor imager and GST-AMPKα-1–392 and α-SNAP were examined by immunoblotting. (c)32P phosphate release was measured by scintillation counting and specific activity of different amounts of α-SNAP calculated. (d) Phosphorylated FLAG-AMPKα2 was purified from activated HEK293T cells and incubated for 30 min with GST (as control, CON), or α-SNAP WT, M105I, L294A or 1–285 (0.5 μg each). Phosphorylated T172 of AMPKα2 was analysed by immunoblotting. (e) Raptor and Akt were expressed in HEK293T cells, purified by FLAG or MYC immunoprecipitation and incubated with GST (as control, CON), or α-SNAP WT, M105I, L294A or 1–285 (0.5 μg each). Phosphorylation of Akt T308 and Raptor S792 were analysed by immunoblotting. Figure 4: α-SNAP dephosphorylates pT172 in AMPKα. ( a ) Coomassie blue staining of purified wild-type (WT) α-SNAP, mutants M105I, L294A and 1–285 were purified, used in assays for phosphatase activity. ( b , c ) 32 P-labeled GST-AMPKα1–392 recombinant protein was used as substrate of α-SNAP phosphatase. α-SNAP (2, 5, 10 and 50 ng) was incubated with 32 P-GST-AMPKα-1–392. ( b ) 32 P-GST-AMPKα-1–392 recovered by trichloroacetic acid precipitation was resolved in SDS–PAGE and detected by phosphor imager and GST-AMPKα-1–392 and α-SNAP were examined by immunoblotting. ( c ) 32 P phosphate release was measured by scintillation counting and specific activity of different amounts of α-SNAP calculated. ( d ) Phosphorylated FLAG-AMPKα2 was purified from activated HEK293T cells and incubated for 30 min with GST (as control, CON), or α-SNAP WT, M105I, L294A or 1–285 (0.5 μg each). Phosphorylated T172 of AMPKα2 was analysed by immunoblotting. ( e ) Raptor and Akt were expressed in HEK293T cells, purified by FLAG or MYC immunoprecipitation and incubated with GST (as control, CON), or α-SNAP WT, M105I, L294A or 1–285 (0.5 μg each). Phosphorylation of Akt T308 and Raptor S792 were analysed by immunoblotting. Full size image Effects of overexpression of WT and α-SNAP mutants L294A and 1–285 in cells Overexpression of WT α-SNAP reduced basal phosphorylation of T172 in AMPK in unstimulated cells and significantly reduced activation of AMPK and downstream signalling to S79 in ACC in response to addition of 2-deoxyglucose to the cells ( Fig. 5a ). In contrast, expression of the same levels of the L294A or 1–285 forms of α-SNAP did not significantly reduce the basal level of T172 phosphorylation or affect the activation in response to addition of 2-deoxyglucose to the cells ( Fig. 5a ). Moreover, only the WT α-SNAP, but not the L294A or 1–285 forms, rescued cells from α-SNAP knockdown, in terms of increased AMPK, ACC and Raptor phosphorylation ( Fig. 5b ). The significant increase in mitochondrial biogenesis due to knockdown of α-SNAP, measured by citrate synthase activity, was prevented by overexpression of WT, but not by L294A or 1–285 forms of α-SNAP ( Fig. 5c ). The HA-tagged L294A and 1–285 mutated α-SNAPs co-immunoprecipitated the FLAG-tagged α subunit of AMPK comparable to WT α-SNAP, indicating the mutations in the C-terminal region of the protein did not eliminate binding to AMPK ( Fig. 5d ). The results suggest that the negative regulation of AMPK by α-SNAP in living cells was not simply because of protein–protein association, but probably depended on the phosphatase activity of α-SNAP. 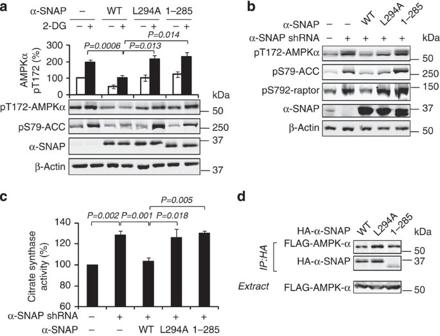Figure 5: Effects of α-SNAP mutations on inactivation of AMPK. (a) The α-SNAP WT, L294A and 1–285 proteins were expressed in HEK293T cells that were treated (−/+) 25 mM 2-DG. Data represent mean±s.e.m. forn=3 and statistical analysis of pairedt-test was performed. (b) HEK293 cells were infected with lentiviral shRNA targeting GFP (as control) or α-SNAP (SNAP sh1), followed by expression of α-SNAP WT, L294A and 1–285, as indicated. (c) Citrate synthase activity was measured in the cells prepared as in (b). Data represent mean±s.e.m. (n=4) andP-values from Student’st-test of significance are indicated. (d) FLAG-AMPKα2 and γ1 were co-expressed with HA-α-SNAP WT, L294A and 1–285 in HEK293T cells as indicated. HA immunoprecipitates from cell extracts were analysed by immunoblotting. Figure 5: Effects of α-SNAP mutations on inactivation of AMPK. ( a ) The α-SNAP WT, L294A and 1–285 proteins were expressed in HEK293T cells that were treated (−/+) 25 mM 2-DG. Data represent mean±s.e.m. for n =3 and statistical analysis of paired t- test was performed. ( b ) HEK293 cells were infected with lentiviral shRNA targeting GFP (as control) or α-SNAP (SNAP sh1), followed by expression of α-SNAP WT, L294A and 1–285, as indicated. ( c ) Citrate synthase activity was measured in the cells prepared as in ( b ). Data represent mean±s.e.m. ( n =4) and P- values from Student’s t -test of significance are indicated. ( d ) FLAG-AMPKα2 and γ1 were co-expressed with HA-α-SNAP WT, L294A and 1–285 in HEK293T cells as indicated. HA immunoprecipitates from cell extracts were analysed by immunoblotting. Full size image Evidence for gain-of-function by hyh mutant α-SNAP M105I The hyh (hydrocephalus with hop gait) mouse has structural and behavioural defects and abnormal localization of apical proteins in neuroepithelial cells, attributed to the homozygous point mutation Met105Ile (M105I) in α-SNAP [17] . The mechanistic basis for the hyh phenotype has been an unsolved mystery for over a decade. This single residue substitution was shown to not alter α-SNAP binding to NSF, or NSF-mediated disassembly of SNARE complexes [17] . LKB1 and AMPK have been assigned a role in establishing cell polarity [18] , [19] , and this raised the possibility that the M105I mutation in α-SNAP might produce the hyh phenotype by affecting AMPK. Overexpression of α-SNAP (M105I) was more effective than equivalent levels of WT α-SNAP in preventing AMPK activation and phosphorylation of its substrates ACC and Raptor in response to addition of 2-deoxyglucose to the cells ( Fig. 6a ). This was manifested over a range of 2-deoxyglucose concentrations, where the M105I was consistently more effective than WT α-SNAP at reducing the level of T172 phosphorylation of AMPK ( Fig. 6b ). Furthermore, we observed a significant, ~2-fold increase in M105I α-SNAP co-immunoprecipitation with AMPKα compared with WT α-SNAP ( Fig. 6c ). These data suggest the hyh mutation in α-SNAP is a gain-of-function substitution that enhances binding to AMPK to reduce LKB1-AMPK signalling. However, whether lower AMPK activity is involved in the hyh phenotype merits further investigation. 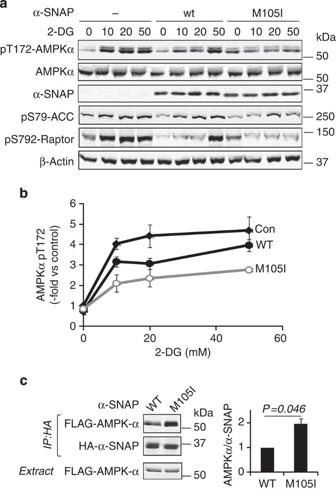Figure 6: Gain-of-function by α-SNAP hyh mutant M105I in binding and inactivation of AMPK. (a) Vector control, α-SNAP WT and M105I were expressed in HEK293T cells. Cells were treated with 10, 20 and 50 mM 2-DG. Cell extracts were analysed by immunoblotting. (b) Quantification of (a). Data represent mean±s.e.m. for three independent experiments. (c) FLAG-AMPKα2 and γ1 were co-expressed with HA-α-SNAP WT or M105I in HEK293T cells. HA immunoprecipitation was performed with cell extract. Data represent mean±s.e.m. (n=3). Figure 6: Gain-of-function by α-SNAP hyh mutant M105I in binding and inactivation of AMPK. ( a ) Vector control, α-SNAP WT and M105I were expressed in HEK293T cells. Cells were treated with 10, 20 and 50 mM 2-DG. Cell extracts were analysed by immunoblotting. ( b ) Quantification of ( a ). Data represent mean±s.e.m. for three independent experiments. ( c ) FLAG-AMPKα2 and γ1 were co-expressed with HA-α-SNAP WT or M105I in HEK293T cells. HA immunoprecipitation was performed with cell extract. Data represent mean±s.e.m. ( n =3). Full size image Our studies reveal α-SNAP as a negative regulator of pT172 in AMPK, limiting activation of the kinase in response to various stimuli, and thereby restricting AMPK suppression of anabolic signalling and induction of mitochondrial biogenesis. We demonstrate direct binding of α-SNAP to AMPK that is affected by ATP, making the binding potentially sensitive to the adenylate energy charge in cells. This is consistent with previous reports of adenine nucleotide effects on AMPK dephosphorylation [8] , [9] . As recombinant α-SNAP in vitro dephosphorylated GST-AMPK we favour a model wherein α-SNAP acts as an AMPK phosphatase in cells, but it is possible other protein phosphatases also are involved in control of AMPK. Okadaic acid, an inhibitor of all the PPP family phosphatases (for example, PP1, PP2A, PP4, PP5, PP6), did not alter basal AMPK activity in rat hepatocytes, arguing against PPPs as AMPK phosphatases [20] . However, okadaic acid was reported to attenuate palmitate-induced inhibition of AMPK activity [21] . Previous results using RNAi suggested that PP1α and PP1β, or PP2A, both of the PPP family, or PPM1E/F of a different phosphatase family could affect pT172 in AMPKα [21] , [22] , [23] . Recent genetic results in yeast implicate Sit4 phosphatase (mammalian PP6) and Glc7 (mammalian PP1) in control of SNF1, the yeast homologue of AMPK [24] . We suggest that perhaps multiple phosphatases can act on AMPK, and there may be some specificity of different phosphatases for individual AMPK isoform combinations. The sequence of α-SNAP does not align with any other known Ser/Thr phosphatases. The properties of α-SNAP as a phosphatase distinguish it from the PPP, PPM and FCP/SCP families of phosphatases [25] (unpublished data). Human α-SNAP is related in sequence to γ-SNAP and Sec17 (the yeast homologue), whose 3D structures consists of N-terminal helical repeats, mostly arranged anti-parallel into an extended twisted sheet, and a C-terminal helical bundle folded back against the sheet [26] , [27] . It is curious that the C termini of these proteins are flexible and the last 30 residues of γ-SNAP and the C-terminal residues of Sec17 were not visualized in the crystal structures. These are the regions we show are critical for the phosphatase activity. Investigating the structural basis of α-SNAP as a phosphatase will require additional experimentation. Our studies demonstrate that α-SNAP negatively regulates AMPK activation and thereby could affect cell growth, metabolism, polarity and development. Knockout of α-SNAP in mice is embryonic lethal and α-SNAP has been associated with pathological conditions [28] . Articles published while this work was in progress reported knockdown of α-SNAP provokes apoptosis in epithelial cells [29] and induces p53 and sensitizes HEK293 cells to cisplatin [30] . Interestingly, AMPK activation also is reported to induce p53 accumulation and inhibit cancer cell proliferation [31] . Because of the reports of apoptosis we tested whether RNAi knockdown of α-SNAP activates AMPK by inducing apoptosis. Extended knockdown of α-SNAP did induce caspase activation, shown by an increase of cleaved PARP, and this was blocked by co-treatment with Z-VAD, a caspase inhibitor ( Supplementary Fig. S2a ). There was no effect +/− Z-VAD on activation of AMPK in response to α-SNAP knockdown. In addition, we found other agents that stimulated apoptosis, such as cisplatin, doxorubicin and TRAIL did not elicit an increase in AMPK activity ( Supplementary Fig. S2b ). As α-SNAP knockdown activates AMPK, maybe AMPK is involved in induction of p53. The effects of α-SNAP knockdown on apoptosis and p53 were proposed to be independent of NSF, the canonical partner of α-SNAP [29] , [30] . We also found that effects of α-SNAP on AMPK did not seem to depend on or involve NSF, so a re-evaluation of the function of α-SNAP in cells seems to be warranted. Our discovery of in vitro phosphatase activity by recombinant α-SNAP WT, but not the previously known inactive L294A and 1–285 forms, suggests a broader repertoire of possible biological functions for this protein, long thought to merely act as an adapter. Whether there are other substrates of the α-SNAP phosphatase besides AMPK or whether α-SNAP serves as an adapter to direct AMPK to phosphorylate substrates are possibilities that deserve further study. We expect our finding of a physical and functional relationship between α-SNAP and AMPK provides interconnections between signalling pathways and intracellular processes that will impact systems biology analyses of network relationships. Antibodies and reagents The antibodies were obtained from the following sources: AMPKα1/2, β1/2, pAMPKα T172, pACC S79, pRaptor S792, pS6K T389, cleaved PARP, NSF and COXIV from Cell Signalling Technology, FLAG, FLAG-M2 bead, HA and β-actin from Sigma, α-SNAP from Exalpha Biologicals, pAkt T308 from Merck, CV-α and CIII-core2 from Mitosciences. Other reagents obtained: Ni-NTA agarose from Qiagen, 2-deoxyglucose, phenformin, oligomycin, ATP, AMP, ATP-γ-S, PNP-AMP, FCCP and rotenone from Sigma, microcystin-LR, okadaic acid, calyculin A and protease inhibitor cocktail from Calbiochem, Z-VAD-fmk from MP Biomedical, Citrate synthase activity assay kit from Sigma, protein G agarose, DiFMUP, Lipofectamine 2,000 and all reagents for cell culture from Invitrogen, Seahorse assay reagents from Seahorse Biosciences, purified PP2A from Merck (Upstate). Other chemicals were from Fisher Scientific. Plasmids The constructs of AMPKα2, β1 and γ1 were gifts from B. E. Kemp (University of Melbourne). α-SNAP human cDNA was obtained from Open Biosystems. The cDNAs of AMPK α2, β1, γ1 and α-SNAP were amplified by PCR and subcloned into epitope tagged vectors by standard protocols. AMPKα2, β1 and γ1 were fused with FLAG tag at N-terminus in pCMV tag-2B. α-SNAP was inserted into pcDNA3 with HA tag at C-terminus and bacterial expression vector pET28a with His tag at N-terminus. Site‐directed mutagenesis (AMPKγ1 R299G, α-SNAP M105I and L294A) was performed using Quick Change II XL (Stratagene) according to the manufacturer’s instructions. α-SNAP truncation from amino acid 1 to 285 (1–285) was obtained by PCR. Cell culture and transfection HEK293, HEK293T and Madin–Darby Canine Kidney cells were cultured in Dulbecco’s modified Eagle’s medium containing 10% foetal bovine serum (FBS). HEK293T or HEK293 cells were seeded in 6-well plate, 6-cm dish and 10-cm dish. Eighteen hours later plasmids were transfected using Lipofectamine 2,000 at 1:1~3 ratio (plasmid:lipofectamine). The cells were harvested and analysed at 36 h after transfection. For stable transfection, cells were selected by G418 with concentration up to 1.5 mg ml −1 and maintained in 80 μg ml −1 of G418 after stable selection. For analysing AMPK activity with α-SNAP, HEK293T cells were grown in Dulbecco’s modified Eagle’s medium containing 5% FBS, 2 mM sodium pyruvate, 5 mM MgCl 2 and 50 mM glucose for 16 h to keep low basal AMPK activity. Cells were treated in this medium containing 5 mM glucose. Cell extract and immunoprecipitation Cells were rinsed once with chilled phosphate-buffered saline (145 mM NaCl, 5.4 mM KCl and 10 mM sodium phosphate,15 mM glucose, pH 7.4) and then scraped and homogenized by repeated passage through a 20-gauge needle. Homogenization buffer contained 25 mM HEPES, pH 7.4, 50 mM β-glycerophosphate, 10 mM sodium phosphate, 10 mM NaF, 2 mM EDTA, 2 mM EGTA, 1 mM dithiothreitol, 0.2% Tween-20 supplemented with 0.5 μM microcystin-LR and protease inhibitor cocktail. Homogenates were centrifuged at 12,000 g for 10 min, and the supernatants were retained for analyses. For immunoblotting, samples were resolved by SDS–PAGE, transferred into nitrocellulose membrane and quantified with an Odyssey fluorescence scanner (Licor Industries) after immunoblotting. For immunoprecipitation, cell extracts (800 μl for 10-cm dish) were incubated with antibodies (2 μg) bound to protein G-agarose beads (10 μl) at room temperature for 1.5 h with constant mixing. The beads were then washed four times with homogenization buffer. Lentiviral shRNA Oligonucleotides encoding the shRNA were annealed and subcloned into pLKO.1 (no. 8453, Addgene). HEK293LT cells (6-cm dish) were co-transfected with 2 μg of plasmids expressing shRNA, 1.5 μg of pCMV-dR8.2dvpr, and 0.5 μg pCMV-VSV-G plasmids using Lipofectamine 2,000. Virus-containing supernatants were collected and combined from 36 to 60 h after transfection and used to infect cells in the presence of 8 μg ml −1 polybrene (Sigma). Infected cells were selected with 4 μg ml −1 puromycin (Sigma) and analysed on the 4–8th day after infection. Mass spectrometry Samples were separated by SDS–PAGE with 6–12.5% gradient gel and visualized by silver staining. Protein bands were excised and protein identification was performed at the Vincent Coates Foundation Mass Spectrometry Laboratory, Stanford University. After in-gel trypsin digestion, trypsin-generated peptides were analysed by liquid chromatography-coupled tandem mass spectrometry/mass spectrometry. Proteins were identified by comparing the mass spectrometry data against the NCBInr protein database through the Mascot search engine. Purification of recombinant proteins His-tagged forms of α-SNAP wild-type (WT), M105I, L294A and 1-285 and GST-tagged AMPKα 1–392 were expressed in Escherichia coli BL21 -RIPL and purified. Briefly, 1 l cultures were grown at 37 °C for 12–16 h to A 600 =1.5 and induced with 0.1 mM isopropyl-1-thio-β-D-galactopyranoside at 14 °C for 20–24 h. Bacterial pellets collected by centrifugation were resuspended in lysis buffer (20 mM Tris, 100 mM NaCl, 1 mM phenylmethylsulfonyl fluoride, 10 mM imidazole, 0.5% Triton X-100, pH 8.0). Cells were broken by freeze-thaw for 2 cycles and sonicated (60 s), and lysates were centrifuged for 20 min at 4,000 g . α-SNAP was purified from the supernatant by binding to Ni-NTA agarose and elution with imidazole (200 mM). Proteins were dialyzed against buffer (20 mM Tris, 100 mM NaCl, 1 mM dithiothreitol, pH 7.4) for 2–3 times. To assess purity and to confirm protein concentrations, samples were subjected to SDS–PAGE and then stained with Coomassie blue. We found that concentrated solutions of α-SNAP tended to undergo aggregation, with loss of phosphatase activity. After testing a variety of conditions we found that dilution in pH 4.0 buffers with 0.5% lauryldimethylamine oxide provided consistently higher activity. Binding assay of α-SNAP and AMPKγ FLAG-tagged AMPKγ was expressed in HEK 293 T cells and isolated with anti-FLAG antibody coupled to Protein G-Agarose beads. One third of beads was mixed with 1 μg purified recombinant α-SNAP in 100 μl assay buffer (50 mM Tris pH 7.4, 100 mM NaCl, 1 mM DTT, 0.2% Triton X-100 and 1% BSA) supplemented with or without nucleotides, and incubated at room temperature for 20 min. The beads were washed by centrifugation four times with assay buffer and bound proteins analysed by fluorescent immunoblotting and quantification with an Odyssey 2D IR scanner (Licor Industries.). Phosphatase activity assay GST-AMPKα 1–392 recombinant protein was phosphorylated in vitro by CaMKK II (a generous gift from Art Edelman) with 32 P-ATP. The reaction included 50 mM Tris pH 7.4, 1 mM DTT, 10 mM MgSO 4 , 1 mM MnCl 2 , 1 mM CaCl 2 , 10 unit μl −1 calmodulin, 2 mM ATP (200 μCi per mM 32 P-ATP), 2 mg GST-AMPKα 1–392 protein and 10 μg CaMKK II, incubating at 37 °C for 24 h. The reaction was terminated by adding 1/9 volume of 100% TCA, followed by dialysis of precipitated proteins in the buffer of 50 mM Tris pH 7.4, 5 mM DTT and 0.01% Brij 35 for 16 h. Phosphatase assay with phosphoprotein was performed using trichloroacetic acid precipiatation according to the procedure described previously. [1] For in vitro phosphatase assay with AMPK, FLAG-AMPKα2 was expressed in HEK293T cells that were stimulated with 25 mM 2-DG to activate the AMPK. FLAG-M2 beads were used to recover the phosphorylated FLAG-AMPKα2 that was eluted by FLAG peptide (0.5 μg μl −1 ). The purified phosphorylated proteins were incubated for 30 min with 0.5 μg of α-SNAP WT, M105I, L294A, 1–285 recombinant proteins and GST (as control) in assay buffer (50 mM Tris, 1 mM dithiothreitol, 10 mM MgCl 2 , 10 μM ATP, pH 7.4). AMPKα2 pT172 was examined by fluorescent immunoblotting. Measurements of OCR and extracellular acidification rate A Seahorse Bioscience XF24-3 Extracellular Flux Analyser was used to measure OCR and ECAR. HEK293T cells (25,000 cells each well) were seeded in poly- L -lysine coated XF24 cell culture plate for 18–24 h. The media was replaced with XF assay media (143 mM NaCl, 5.4 mM KCl, 0.8 mM MgSO 4 , 1.8 mM CaCl 2 , 0.91 mM NaH 2 PO 4 , 15 mg ml −1 phenol red supplemented with 15 mM glucose, 2 mM sodium pyruvate, 1 mM glutamine and 2% FBS) and equilibrated in non-CO 2 incubator for 1 h. Seahorse analyser uses a cartridge with 24 optical fluorescent O 2 and pH sensors to measure OCR (pmol/min) and ECAR (mPh min −1 ). Basal OCR and ECAR were measured for 3 min every 10 min for four points, followed by sequential injection of oligomycin (3 μM), 2-DG (25 mM), FCCP (1 μM) and Rotenone (1 μM). Each treatment was measured for 3 min every 10 min for 2 points. After measurement of OCR and ECAR, media is removed carefully and completely and 20 μl lysis buffer (20 mM Tris, 0.1% Triton X-100, protease inhibitor cocktail, pH 7.4) was added and protein concentration was analysed to normalize OCR and ECAR. Citrate synthase activity assay HEK293T cells were homogenized in buffer containing 0.2% Tween-20 and 0.1% Triton X-100 and freeze-thawed once. Homogenates were centrifuged at 12,000 g for 10 min, and the supernatants were retained for analyses. Samples of 3 μg protein were used for assay in 96-well microplate. The assay was performed following to manufacturer’s instructions. Plate was read at 412 nm on kinetic programme in linear response range (up to 10 min) and enzyme activity units (μmol min −1 mg −1 protein) calculated from the change in absorbance (ΔA 412 )/min according to the instructions. How to cite this article: Wang, L. and Brautigan, D.L. α−SNAP inhibits AMPK signaling to reduce mitochondrial biogenesis and dephosphorylates Thr172 in AMPKα in vitro . Nat. Commun. 4:1559 doi: 10.1038/ncomms2565 (2013).